Coupling of plasmonic and optical cavity modes in quasi-three-dimensional plasmonic crystals The field of plasmonics has emerged as an interesting area for fundamental studies, with important application possibilities in miniaturized photonic components. Plasmonic crystals are of particular relevance because of large field enhancements and extraordinary transmission that arise from plasmonic interactions between periodic arrays of metallic elements. Here we report methods to enhance and modify the plasmonic resonances in such structures by strongly coupling them to optical modes of Fabry–Perot type cavities. First, we illustrate a type of plasmonic, narrow-band (~15 nm), high-contrast (>20 dB) absorber and an opto-fluidic modulator based on this component. Second, we use optimized samples as substrates to achieve strong amplification (>350%) and modulation (>4×) of surface-enhanced Raman scattering from surface-bound monolayers. Cavity-coupling strategies appear to be useful not only in these two examples, but also in applications of plasmonics for optoelectronics, photovoltaics and related technologies. Surface plasmons are coherent oscillations of electrons at metal-dielectric interfaces that can exist either in localized or propagating forms [1] . Such electromagnetic disturbances can be exploited for wide-ranging applications, from biological and chemical sensors based on changes in near-surface refractive index or Raman scattering [2] , to devices for sub-wavelength manipulation of light [3] , wave-guiding [4] , optical modulation [5] , Bragg reflection [6] , photo detection [7] , [8] , lasers [9] and solar energy generation [10] . Methods to modify plasmonic interactions by controlling the shapes and sizes of the metal structures, [11] , [12] the types of metals [13] , [14] or the indices of refraction of the surrounding materials [2] , [15] are firmly established. Newer approaches integrate plasmonic components into equivalent circuit structures such as metal–insulator–metal stacks [16] , [17] , [18] . Here we report a different strategy in which light transmitted through a quasi-three-dimensional (quasi-3D) plasmonic crystal strongly couples with an underlying, Fabry–Perot cavity. We show that, in certain configurations, this arrangement leads to strongly enhanced or diminished reflections (~23 dB change), due to significant modifications in the nature of the plasmonic modes, in a way that can be tuned reversibly using the techniques of opto-fluidics. Associated amplification in the surface plasmon field can also be exploited, to increase signal levels in surface-enhanced Raman scattering (SERS) experiments, by up to ~350% and to modulate SERS signals (>4×) in ways that are not possible with other known techniques. We capture all of these effects in a quantitative way by finite-difference time-domain (FDTD) electromagnetic modelling and systematic experiments. The design possibilities enabled by these ideas, especially when implemented using simple, large-area soft-imprint lithography techniques, lead to new classes of photonic/plasmonic components. Cavity-coupled plasmonic crystal system The structures are formed by first imprinting a square array of sub-wavelength cylindrical depressions [19] , [20] , [21] on the surface of a thin polymer film cast on a glass substrate coated with a layer of gold. Blanket deposition of a thin layer of gold on the imprinted surface of the polymer completes the fabrication. Here a two-dimensional plasmonic crystal, formed by the top gold coating, optically couples to an array of isolated disks of gold in the bottoms of the cylindrical depressions. Light transmitted through this 'quasi-3D' crystal via plasmonic coupling between the nanoholes and recessed disks [22] coherently reflects from the back mirror (that is, the layer of gold on glass) which in turn, influences the plasmonic resonances, constructively or destructively depending on the cavity length. 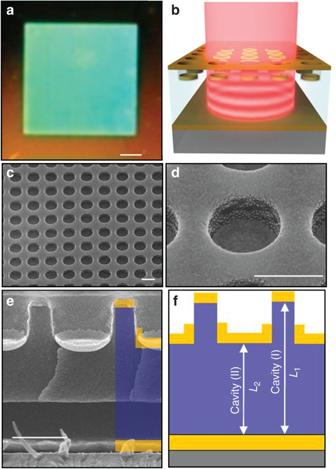Figure 1: Cavity-coupled quasi-3D plasmonic crystal. Large area optical image (scale bar 1 mm) (a) and schematic illustration (b) of a cavity-coupled, quasi-3D plasmonic crystal. Top view SEM (c) of a small region of the sample shown in (a), with magnified view of a unit cell (d). Cross-sectional SEM (e) and schematic illustration (f) of a unit cell showing gold on the raised and recessed regions of the plasmonic crystals, and the gold back reflector for the coupled optical cavities (lengths,L2andL1, as in (e)). Scale bar 500 nm. Figure 1 shows a large area (5 mm×5 mm) optical image ( Fig. 1a ) and a schematic illustration ( Fig. 1b ) of the plasmonic crystal–optical cavity system. A scanning electron microscope (SEM) top view image appears in Figure 1c , along with a magnified view of an individual nanohole/nanodisk ( Fig. 1d ). Figure 1e presents a cross-sectional SEM image and a schematic illustration ( Fig. 1f ) of a unit cell, showing the top gold film with a square lattice of circular holes, recessed circular gold disks (with some gold on the sidewalls near the base) and the gold back reflector ( H BR ). The choice of nanohole period, P =740 nm, and diameter, D =500 nm, maximizes the strengths of localized surface plasmon resonances (LSPRs) of interest for present purposes [20] . This system embeds two asymmetric Fabry–Perot cavities, both with the thick gold as a back reflector: one formed by the gold in the raised regions of the top surface (Cavity (I)) and the other by the gold in the recessed regions (Cavity (II)). The lengths of these two cavities are related by the depth of moulded relief ( H RD ), as shown in Figure 1f . Figure 1: Cavity-coupled quasi-3D plasmonic crystal. Large area optical image (scale bar 1 mm) ( a ) and schematic illustration ( b ) of a cavity-coupled, quasi-3D plasmonic crystal. Top view SEM ( c ) of a small region of the sample shown in ( a ), with magnified view of a unit cell ( d ). Cross-sectional SEM ( e ) and schematic illustration ( f ) of a unit cell showing gold on the raised and recessed regions of the plasmonic crystals, and the gold back reflector for the coupled optical cavities (lengths, L 2 and L 1 , as in ( e )). Scale bar 500 nm. Full size image The geometries of the depressions, the thicknesses of the gold layers and the indices of the surrounding dielectric media (air and polymer) define the wavelengths of the LSPRs. The optical cavities strongly modify these resonances. 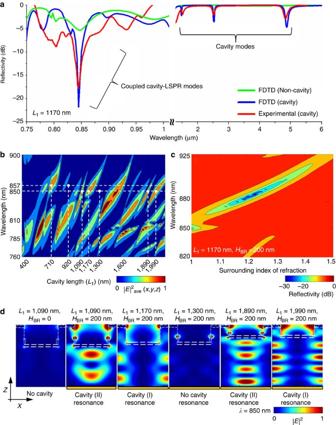Figure 2: Measured and computed properties in a cavity-coupled quasi-3D plasmonic crystal. (a) Measured and FDTD-computed far-field reflectivity of a cavity-coupled plasmonic crystal system having cavity lengthL1=1,170 nm with a thick back reflectorHBR=200 nm. Calculation for the case ofHBR=0 nm is also shown. (b) FDTD-computed variation of the intensity (|Ē|2), spatially averaged across a conformal surface located 10 nm above the top and bottom Au layers, as a function of cavity length (L1) and wavelength. (c) FDTD-computed variation of the far-field reflectivity as a function of surrounding medium refractive index forL1=1,170 nm. (d) FDTD-computed cross-sectional (X–Z) intensity distributions across a unit cell for various configurations. The results clearly show the influence of both cavities in this system. Figure 2a shows the far-field reflectivity spectra measured experimentally and computed by FDTD, for a cavity-coupled plasmonic crystal with L 1 =1,170 nm and H BR =200 nm, along with FDTD results for a case without the cavity (that is, H BR =0 nm). The cavity clearly enhances the LSPR resonance that appears in the wavelength range 780–900 nm, as manifested by a strong, sharp dip in the reflection at ~845 nm. The long-wavelength region (1.5–6 μm), which lies away from the plasmonic resonances, shows unmodulated cavity modes, due to the combined effects of Cavity (I) and Cavity (II) ( Supplementary Fig. S1 ). To reveal further features, Figure 2b shows computed variations in the electric field intensity (| Ē | 2 ) spatially averaged across a conformal surface that extends over a unit cell of the plasmonic crystal at a position 10 nm above the raised and recessed regions of the gold layers, as a function of cavity length ( L 1 ) and the excitation wavelength, with all other structure parameters fixed, except for L 2 , which changes according to L 2 = L 1 − H RD . The results show that the plasmon resonances bend and repeat with changes in L 1 , as they come into and out of overlap with the cavity modes ( Supplementary Figs S2 and S3 ). As might be expected, the cavity length and refractive index of the dielectric layer influence the effective optical-path lengths and, therefore, the positions of the cavity-mode resonances. By contrast, the index of the surroundings predominantly affects only the plasmonic component of the responses. Figure 2c shows the FDTD-computed variation of the far-field reflection as a function of this index, for a structure with L 1 =1,170 nm. Here the LSPR, initially near 850 nm, moves to higher wavelengths with increasing index, hence reducing field enhancements due to de-tuning away from the cavity resonance. The phenomenon repeats because of overlap between the shifted LSPR and another cavity mode at an index of ~1.22 at a wavelength ~885 nm. The nature of the coupling is clearly visible in the cross-sectional intensity distributions of Figure 2d , computed using FDTD for linearly polarized light at a wavelength of 850 nm for air ( n =1) as the surrounding medium. Specifically, the main plasmonic resonance is strongly enhanced when L 1 is 1,170 or 1,990 nm and when L 1 is 1,090 or 1,890 nm, due to the presence of standing waves (that is, cavity modes) corresponding to the action of Cavity (I) and Cavity (II), respectively. For reference, when L 1 =1,300 nm, no cavity mode is present and no enhancement results. The cross-sectional intensity distribution for H BR =0 (that is, non-cavity case) at L 1 =1,090 nm provides further evidence of the importance of the cavity ( Supplementary Fig. S2 ). Figure 2: Measured and computed properties in a cavity-coupled quasi-3D plasmonic crystal. ( a ) Measured and FDTD-computed far-field reflectivity of a cavity-coupled plasmonic crystal system having cavity length L 1 =1,170 nm with a thick back reflector H BR =200 nm. Calculation for the case of H BR =0 nm is also shown. ( b ) FDTD-computed variation of the intensity (| Ē | 2 ), spatially averaged across a conformal surface located 10 nm above the top and bottom Au layers, as a function of cavity length ( L 1 ) and wavelength. ( c ) FDTD-computed variation of the far-field reflectivity as a function of surrounding medium refractive index for L 1 =1,170 nm. ( d ) FDTD-computed cross-sectional ( X – Z ) intensity distributions across a unit cell for various configurations. The results clearly show the influence of both cavities in this system. Full size image Narrow-band plasmonic absorber/filter and opto-fluidic modulator There are several ways to exploit the behaviours illustrated in Figure 2 . The physics that governs the responses of these structures is different than that associated with absorbers that use other types of plasmonic structures and metamaterials [23] , [24] , [25] . The remarkably strong absorption and narrow-band operation reported here represent appealing features for applications in tunable filters, substrates for SERS, and other devices, as described in the following. In a first example, we demonstrate a class of narrow-band absorber, or reflective notch filter, and a modulator based on this component. The underlying effect is that light can be either nearly completely absorbed or completely reflected, depending on cavity lengths, by virtue of cavity controlled excitation of LSPRs on the gold surfaces. 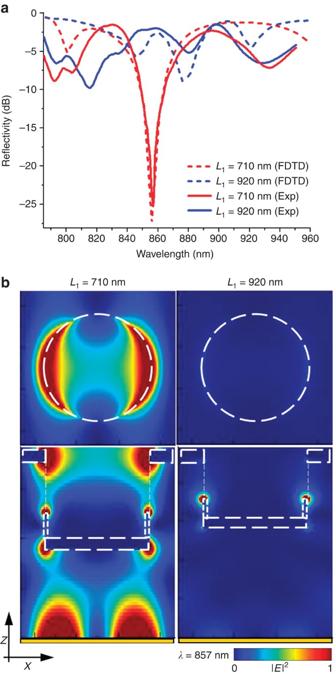Figure 3: Cavity controlled narrow-band absorption in a plasmonic crystal. (a) Far-field reflection as a function of wavelength measured and computed (FDTD) from structures for cavity lengths ofL1=710 nm (Absorption ON) andL1=920 nm (Absorption OFF), both with a back reflector thickness ofHBR=200 nm. (b) FDTD-computed top (X–Y) and cross-sectional (X–Z) intensity distributions for these two cases, atλ=857 nm. Figure 3a shows the variation of far-field reflection as a function of wavelength for L 1 =710 nm and 920 nm. The former configuration results in an enhanced plasmonic resonance and low far-field reflection, which we label as the 'Absorption ON' state. The latter corresponds to a suppressed plasmonic resonance and high far-field reflection, that is 'Absorption OFF'. Coupling between LSPR modes and standing waves in the Fabry–Perot cavity originates from coherent interference effects. When the cavity produces constructive (destructive) interference near the surface of the structure, the fields available to excite LSPR modes are maximized (minimized), and the resonance is thereby enhanced (suppressed). For example, when L 1 =710 nm, the round trip phase delay from propagation in the cavity is ~4 π for the wavelength, λ =857 nm, that coincides with the main LSPR. In this scenario, constructive interference occurs, thereby enhancing the LSPR. Similarly, for L 1 =920 nm, the phase delay is ~5 π , destructive interference obtains, and the LSPR is suppressed. These outcomes are apparent in the results of Figure 3a , where the transmission dip associated with the LSPR is large and small for L 1 =710 nm and 920 nm, respectively. The measured bandwidth (15 nm, FWHM) and depth of the resonant dip in reflection at λ =857 nm closely match FDTD predictions. Figure 3b shows top (X–Y) and cross-sectional (X–Z) views of the intensity distributions. The 'Absorption ON' case shows a complex coupled Cavity (II) type mode, whereas the 'Absorption OFF' configuration indicates an absence of cavity effects. These two states also appear in characteristic features of Figure 2b (white vertical dashed lines on the left, at L 1 =710 and 920 nm). This structure, then, represents an unusual optical component, with absorption properties that can be designed by appropriate choice of cavity dimensions. The position of the plasmonic absorption band depends strongly on the geometry of the plasmonic crystal (for example, P, D) [9] and the intrinsic properties of the gold. Alternative metals can provide further flexibility in design [13] . When viewed as a reflective filter, the extinction coefficient (>−25 dB) and bandwidth (~15 nm) of this three-layer plasmonic device are comparable to parameters that require, in a multilayer dielectric thin film Bragg structures, at least 20 alternating quarter-wave stacks with low index contrast (Δ n ~0.05–0.1) plus a half-wave defect layer followed by another 20-layer quarter wave stack [26] . Figure 3: Cavity controlled narrow-band absorption in a plasmonic crystal. ( a ) Far-field reflection as a function of wavelength measured and computed (FDTD) from structures for cavity lengths of L 1 =710 nm (Absorption ON) and L 1 =920 nm (Absorption OFF), both with a back reflector thickness of H BR =200 nm. ( b ) FDTD-computed top ( X – Y ) and cross-sectional ( X – Z ) intensity distributions for these two cases, at λ =857 nm. Full size image An extra attractive aspect of this type of cavity-coupled plasmonic component is that its properties can be tuned, dynamically, by changing either the dimensions or index of refraction of the cavity. For example, adjusting the cavity index by amounts (~5–10%) achievable with organic electro-optic materials [27] can accomplish complete switching ( Supplementary Fig. S4 ). An alternative, and simpler, mode of tuning involves changing the surrounding refractive index, using effects summarized in Figure 2c . 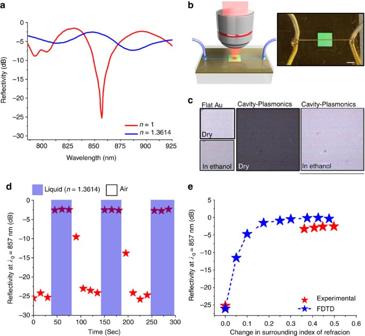Figure 4: Narrow band plasmonic absorber/filter and opto-fluidic modulator. (a) Switching 'ON' and 'OFF' of reflectivity due to shifts in the LSPR by a contacting liquid (n=1.36) on the top gold surface. (b) Moulded Opto-fluidic chip mounted on a cavity-coupled plasmonic crystal; (left) schematic and (right) actual fabricated system. (c) Optical images of this cavity-coupled plasmonic crystal system in air and immersed in ethanol collected in reflection mode through a narrow band bandpass filter (815–885 nm). (d) Opto-fluidic switch showing a large change in reflectivity; measured reflectivity as a function of refractive index atλ0=857 nm is shown in (e). Scale bar 2.5 mm. Figure 4a shows, as a demonstration, reflection spectra collected from a sample with L 1 =710 nm, switched between ON (−25 dB) and OFF (2 dB) states at λ 0 =857 nm by replacing the surrounding air with ethanol ( n =1.3614). The techniques of opto-fluidics allow this type of switching to be achieved in an integrated manner. Figure 4b shows a schematic illustration (left) and picture (right) of a device consisting of micro channel created by the contact of an embossed elastomer against a substrate that supports a cavity-coupled plasmonic structure. Optical images of this plasmonic crystal system in air and immersed in ethanol, collected in reflection mode through a narrow band bandpass filter (815–885 nm), appear in Figure 4c . Significant changes in brightness correspond to large differences in reflectivity between the air and ethanol cases. These changes occur uniformly over the entire imaged area, as expected based on the high quality of samples formed by soft imprint lithography procedures. Using a syringe pump, the surrounding material can be switched from ethanol to air, and back again, in a reversible manner. Here the LSPR, initially near 857 nm, moves to higher wavelengths because of the increased index of the surroundings. As a result, the LSPR and cavity modes are no longer in resonance, thereby eliminating the enhancement effects. The process operates in a reversible manner such that the reflectivity goes down to its original value as the surrounding medium is switched from ethanol back to air, as shown in Figure 4d . The same channel system allows more systematic study with different liquids having refractive indices between 1.36–1.5. The change in reflectivity at λ 0 =857 nm as a function of refractive index appears in Figure 4e ; FDTD results indicate a linear variation with index up to ~Δ n =0.15, after which the absorption saturates to its OFF-state value. Figure 4: Narrow band plasmonic absorber/filter and opto-fluidic modulator. ( a ) Switching 'ON' and 'OFF' of reflectivity due to shifts in the LSPR by a contacting liquid ( n =1.36) on the top gold surface. ( b ) Moulded Opto-fluidic chip mounted on a cavity-coupled plasmonic crystal; (left) schematic and (right) actual fabricated system. ( c ) Optical images of this cavity-coupled plasmonic crystal system in air and immersed in ethanol collected in reflection mode through a narrow band bandpass filter (815–885 nm). ( d ) Opto-fluidic switch showing a large change in reflectivity; measured reflectivity as a function of refractive index at λ 0 =857 nm is shown in ( e ). Scale bar 2.5 mm. Full size image Cavity-induced enhancement and deep modulation of SERS In a different application example, the enhanced field strengths associated with cavity-coupled plasmonics ( Fig. 2b ) can be exploited to improve performance in SERS-based sensors. To demonstrate this possibility, we examined scattering from a monolayer of benzenethiol formed on samples like the one of Figure 1c , using linearly polarized excitation light at λ Ex =785 nm. 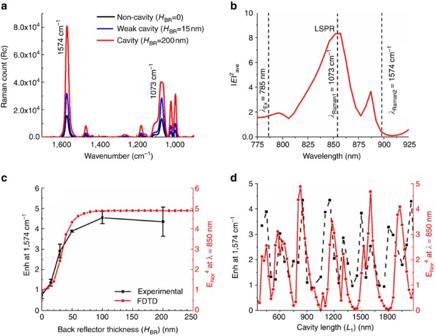Figure 5: Enhancement and modulation of Raman signal. (a) Measured Raman spectra for non-cavity (HBR=0) and cavity (HBR=15 and 200 nm) configurations of quasi-3D plasmonic crystals. The two main peaks observed here,λRaman1andλRaman2, are characteristic of benzenethiol. (b) Corresponding FDTD-computed intensity, |E|2ave, averaged across a conformal surface located 10 nm above the top and bottom Au layers, for a back reflector thickness ofHBR=200 nm and cavity lengthL1=850 nm (all other parameters remained same). The dominant peak is due to an LSPR. The locations of the laser excitation and Raman peaks are marked asλEx,λRaman1andλRaman2respectively. (c) Measured variation of the Raman enhancement atλRaman2=1,574 cm−1and corresponding FDTD-computed normalized, and spatially averaged, squared intensity (ENor4), both as a function of back reflector thickness. (d) Plot similar to the one in (c), but plotted as a function of cavity length. Figure 5a shows measured 'Raman counts' (Rc) for 3 cases, all with L 1 =850 nm, but with 3 different values for H BR : 0, 15 and 200 nm. The spectra show expected signatures for benzenethiol, but with signal enhancements, defined as Enh( L 1 , H BR )=Rc( L 1 , H BR )/Rc( L 1 , H BR =0), of ~350% and ~200% for the bands at 1,574 and 1,073 cm −1 , respectively. This outcome is consistent with the physics summarized in Figure 2 . Figure 5b shows the average intensity computed by FDTD on a conformal surface 10 nm above top and bottom Au layer for H BR =200 nm and L 1 =850 nm, where benzenethiol is considered as the surrounding medium. The dominant local maximum observed in this plot is identified as an LSPR. The wavelengths of the Raman peaks are λ Raman1 =857 nm and λ Raman2 =896 nm. The LSPR resonance ( λ LSPR ) spans across wavelengths that lie halfway between λ Ex and λ Raman , for both peaks, thereby simultaneously satisfying the approximate requirement ( λ LSPR ≈( λ Ex + λ Raman )/2) for maximum SERS enhancement [1] , [28] , [29] . Figure 5c shows the measured variation of enhanced Raman counts at λ Raman2 , as a function of H BR , together with FDTD-computed values of normalized field intensity squared ( E Nor 4 ) where E Nor =| E ave BR |/| E ave BR=0 |, spatially averaged at 10 nm away from the surfaces, as in the other cases, at a wavelength of 850 nm, normalized to a structure with H BR =0, all with L 1 =850 nm. The experimental and FDTD results show remarkably good agreement, thereby providing confirmation of the cavity-related physics and origins of SERS signals. Figure 5: Enhancement and modulation of Raman signal. ( a ) Measured Raman spectra for non-cavity ( H BR =0) and cavity ( H BR =15 and 200 nm) configurations of quasi-3D plasmonic crystals. The two main peaks observed here, λ Raman1 and λ Raman2 , are characteristic of benzenethiol. ( b ) Corresponding FDTD-computed intensity, | E | 2 ave , averaged across a conformal surface located 10 nm above the top and bottom Au layers, for a back reflector thickness of H BR =200 nm and cavity length L 1 =850 nm (all other parameters remained same). The dominant peak is due to an LSPR. The locations of the laser excitation and Raman peaks are marked as λ Ex, λ Raman1 and λ Raman2 respectively. ( c ) Measured variation of the Raman enhancement at λ Raman2 =1,574 cm −1 and corresponding FDTD-computed normalized, and spatially averaged, squared intensity ( E Nor 4 ), both as a function of back reflector thickness. ( d ) Plot similar to the one in ( c ), but plotted as a function of cavity length. Full size image The plasmon resonances can be constructively or destructively influenced by cavity modes. Figure 5d shows the result of this effect on the SERS measurement, in which the enhancement in Raman counts for λ Raman2 appears as a function of cavity length for constant H BR =200 nm. As with Figure 5c , the Raman counts and FDTD-computed average values of | E | 4 , again normalized to the case where H BR =0, exhibit good agreement. The results show SERS signals that follow cavity-coupling effects discussed previously in the context of Figure 2b . The ability to control the response over a range of >4×, including strong amplification (that is, 350% increase) by adjusting only the cavity length is a notable outcome of the physics. Further optimized structures and materials offer promise for achieving even larger effects. This collective set of results indicates that simple strategies for coupling optical cavities to plasmonic modes can induce responses with practical interest in photonics and sensing. The out-of-plane cavities and the quasi-3D plasmonic crystals presented here are not the only types of structures that can be configured in this way. Arrays of metallic particles, waveguide resonators, in-plane cavities and many other possibilities also appear interesting to consider. A broad consideration of these layouts, together with other materials, in homogeneous or heterogeneous configurations, represent directions for future work. Plasmonic cavity fabrication Large area (5 mm×5 mm) square arrays of sub-wavelength cylindrical depressions were moulded onto the surface of a thin layer of a photo curable epoxy (SU8, MicroChem), using the techniques of solvent-assisted soft imprint lithography, wherein a small amount of ethanol was used to wet the epoxy surface before pressing the substrate against a poly(dimethylsiloxane) (PDMS, 10:1 Sylgard 184) mould containing the inverse pattern. The thickness of the epoxy was controlled through dilution of SU8 photoresist in cyclopentanol and conditions for the spin-coating process. A gold-coated glass substrate served as the substrate. Blanket deposition of a thin layer of gold (~50 nm) by electron beam evaporation completed the fabrication process. Opto-fluidic system The opto-fluidic system was created with a piece of a PDMS with suitable structures of relief on its surface, formed by casting and curing against a pattern of photoresist on a silicon wafer. Contacting the PDMS against a substrate that supports a cavity-coupled plasmonic crystal led to the formation of a liquid-tight seal, thereby establishing a microfluidic channel. Liquid was injected into the channel, through tubes inserted into inlets machined through the thickness of the PDMS, using a syringe pump. For refractive index sensing, we used ethanol ( n =1.3614), tetrahydrofuran ( n =1.4072), chloroform ( n =1.4458) and toluene ( n =1.4969). FDTD model The detailed FDTD model of the actual structure of Figure 1e appears in Supplementary Figure S5 where Cavity (I) and Cavity (II) lengths are L 1 , L 2 and the back reflector, top and bottom gold layer, relief depth, side wall height and thicknesses are H BR , H top , H bottom , H RD , H sidewall and t sidewall , respectively. A Drude plus two-pole Lorentzian model for the complex frequency-dependent gold permittivity was employed, with parameters fit to empirical dielectric constant data [30] . The structure was excited with linearly polarized, plane-wave light. Here we used FDTD to 'fit' our transmission data as shown in Supplementary Figure S6 , and then used that model, with those fitted parameters, to explore various trends and effects with cavity length, index and back reflector thicknesses. To establish correspondence between experiment and modelling ( Supplementary Fig. S5 ), transmission through two different geometries, one with no back reflector ( H BR =0) and one with a thin back reflector ( H BR =15 nm), were compared, both with L 1 =710 nm and H RD =360 nm. We then varied H top between 45–55 nm, H bottom between 45–55 nm, H sidewall between 90–120 nm, and t sidewall between 10–25 nm, in an iterative fashion, to yield a good match between experiment and modelling. The best fit was found for constant L 1 =710 nm, H RD =360 nm and H top =50 nm, H bottom =40 nm, H sidewall =100 nm, and t sidewall =15 nm thicknesses. A final optimization was then performed by varying L 1 by ±20 nm to yield a 'best' fit to study the effects of cavity length on LSPR keeping all other parameters constant. In all cases, the magnitudes of variations explored for each parameter were within uncertainties in physical measurements (ellipsometer, SEM). The transmission through the fabricated structure and FDTD model ( Supplementary Fig. S5 ), for two different geometries, one non-cavity geometry having no back reflector ( H BR =0) and the other one with cavity geometry having a thin back reflector ( H BR =15 nm), were compared for constant L 1 =710 nm, H RD =360 nm, H top =50 nm, H bottom =40 nm, H sidewall =100 nm and t sidewall =15 nm. Supplementary Figure S6a,b shows experimental as well as FDTD-predicted 0-th order transmissions of these two structures, respectively. It can be observed that for the given set of experimentally measured thicknesses, FDTD predictions of transmissions through these two structures matches well with experimental observations. To emulate the actual SERS experimental procedures in FDTD simulation, a 5-nm thick Benzenethiol layer was created on nanohole surface and similar mapping of cavity length versus plasmon resonance was computed. As expected, we observed red-shift of plasmon resonances when the sample is coated with Benzenethiol having higher refractive index ( n =1.588) than air. Far-field reflection measurements Reflection spectra were collected using a ×2.5, 0.07 numerical objective on an optical microscope (Hyperion 2000) coupled to a Fourier transform infrared spectrometer (Vertex 70) and outfitted with a spatial aperture having a diameter of 3.75 mm. Reflection spectra were normalized to a silver mirror with 96% reflectivity over the wavelengths examined. Raman measurements Raman spectra were acquired using a confocal Raman microscope (Senterra, Bruker Optics) with a 75-mm focal-length achromatic lens for both illumination and collection, in place of a microscope objective. The diameter of the pinhole aperture was set to 50 μm. For all measurements, the spectral region from 400–1,800 cm −1 was collected with 3–5 cm −1 spectral resolution. The laser power at the sample was 33 mW with a spot size of 95 μm. The acquisition times were 30 s for all measurements. The sample was illuminated with linearly polarized laser light with a wavelength of 785 nm. The laser beam filled an 2 mm region on the back aperture of the achromatic lens, corresponding to an angular incidence of illumination with a numerical aperture of ~0.02. Data processing of Raman spectra was achieved using OPUS 6.5 (Bruker), including background corrections to account for the dark current response and quantum efficiency of the charge-coupled detector device. Wavelength calibration was also accomplished using OPUS 6.5 to adjust the Raman shift using the atomic emission spectrum of mixed neon and argon gases. How to cite this article: Chanda, D. et al . Coupling of plasmonic and optical cavity modes in quasi-three-dimensional plasmonic crystals. Nat. Commun. 2:479 doi: 10.1038/ncomms1487 (2011).